Multilateral benefit-sharing from digital sequence information will support both science and biodiversity conservation 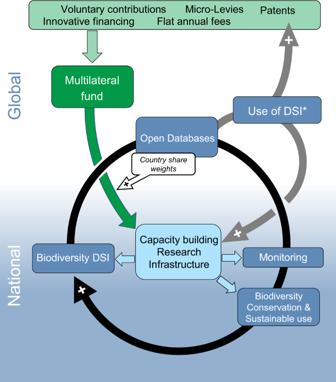Fig. 1: Multilateral funding model for DSI benefit-sharing. Open access to DSI in databases (center blue box) is de-coupled from benefit-sharing (light green box). The multilateral fund (dark green box) can collect funds from micro-levies, voluntary contributions, innovative finance, or from patent royalties. Funding on a national level (dark green arrow) is weighted by the amount of sequences deposited from an individual LMIC, and together with the substantial non-monetary benefit-sharing from DSI (e.g., through international collaborations; lower gray arrow) enables capacity building (especially in the area of genomics and bioinformatics) as well as the build-up of a corresponding research infrastructure. Capacity building improves monitoring, conservation, and sustainable use of biodiversity (dark blue boxes), creating a positive feedback loop that leads to a continuous increase in knowledge generation on biodiversity. Simultaneously, greater availability of DSI creates additional positive feedback loops for generating non-monetary and monetary benefits (gray arrows). The asterisk (*) emphasizes that the use of DSI, and hence the benefits generated, largely depend on the use of DSI originating from several different sources (i.e., countries). Given these pressures, Parties want options. A range of monetary benefit-sharing options for DSI were recently synthesized by the CBD Secretariat [4] . These range from a bilateral system similar to the CBD and its Nagoya Protocol, with access tightly coupled to benefit sharing, to multilateral mechanisms in which access is facilitated through standardized global rules for benefit-sharing. In March 2020, Laird et al. [5] , made a compelling case for multilateralism, and called for the scientific community to work together to develop policy options, but left unanswered what a policy framework could look like. We respond to this call and provide a concrete framework for how DSI benefit-sharing could work (Fig. 1 ). The authors are members of the DSI Scientific Network , a group of scientists from different countries and economic settings that share convergent points of view in the DSI debate. We note that every country provides and uses DSI and, thus, everyone has something to lose and gain [6] . Here, we map out a multilateral framework for DSI that will support biodiversity monitoring and conservation, maintain open access, improve the scientific record, share both non-monetary and monetary benefits, and enable green growth. Fig. 1: Multilateral funding model for DSI benefit-sharing. Open access to DSI in databases (center blue box) is de-coupled from benefit-sharing (light green box). The multilateral fund (dark green box) can collect funds from micro-levies, voluntary contributions, innovative finance, or from patent royalties. Funding on a national level (dark green arrow) is weighted by the amount of sequences deposited from an individual LMIC, and together with the substantial non-monetary benefit-sharing from DSI (e.g., through international collaborations; lower gray arrow) enables capacity building (especially in the area of genomics and bioinformatics) as well as the build-up of a corresponding research infrastructure. Capacity building improves monitoring, conservation, and sustainable use of biodiversity (dark blue boxes), creating a positive feedback loop that leads to a continuous increase in knowledge generation on biodiversity. Simultaneously, greater availability of DSI creates additional positive feedback loops for generating non-monetary and monetary benefits (gray arrows). The asterisk (*) emphasizes that the use of DSI, and hence the benefits generated, largely depend on the use of DSI originating from several different sources (i.e., countries). Full size image The core infrastructure for storing sequence data, the International Nucleotide Sequence Database Collaboration (INSDC) contains 228 million annotated sequences (1.5 billion reads, see https://www.ncbi.nlm.nih.gov/genbank/statistics/ ). The dataset is downloaded partially or completely 34 million times per year, used by more than 10–15 million unique users, and 99.5% of the 750 downstream sequence databases that pull and push DSI through the scientific ecosystem directly rely on the INSDC system [7] . The data are linked to a further 1200 databases and hundreds of thousands of publications that, on average, cite 44 sequences per publication [6] . Clearly, a bilateral system, modelled on the principles of the Nagoya Protocol, that required permission between the end-user and the country of origin for every sequence and user transaction, would be prohibitively complex, affect data interoperability, and be ill-suited for generating knowledge. The DSI statistics above make clear that a human-based system would not work. Technological approaches to track and trace DSI usage would be expensive, complex, and could have a significant environmental footprint. Most importantly, a loss of open access would adversely impact the analytical capacities, data infrastructures, and academic systems in LMICs that rely on these open data infrastructures [2] , [5] , [8] , [9] , [10] and make collaboration with researchers based in countries that enforce DSI use restrictions very unattractive. A bilateral DSI system would also inadvertently create a competitive marketplace that would perversely incentivize the use of DSI from countries where no restrictions exist (e.g., USA, Germany) leading to DSI “forum shopping.” Ironically, DSI from LMICs that are needed most for global monitoring and protection of biodiversity would often be avoided which, in turn, would severely impede progress on the Global Biodiversity Framework. A benefit-sharing framework for DSI clearly needs to be multilateral and should address five fundamental objectives: 1. Open access. Any future benefit-sharing system must guarantee open data access, which is required to be able to use and understand DSI. Only open access enables efficient and broad scale knowledge generation and capacity building. The existing core DSI infrastructure already fulfils these requirements. 2. Simplicity. The DSI data ecosystem is highly complex, even for expert users. For benefit-sharing to happen, the policy framework must be simple. If a complex regulatory layer is added on top of a complex technical system, it is doomed to fail. 3. Harmonize. The DSI dilemma is an opportunity to learn from current inefficiencies in ABS and minimize transaction costs. Furthermore, as DSI is being discussed in multiple international fora, DSI users need a harmonized framework to address benefit-sharing. 4. Biodiversity. Any mechanism needs to effectively support biodiversity conservation and sustainable use (the first two objectives of the CBD). The framework should incentivize and reward biodiversity knowledge generation, and fill in the blank spots on the world map of biodiversity [11] . 5. Fairness. The framework should treat all users and providers fairly and create a level playing field by facilitating both access and compliance evenly across the globe. A multilateral system could nevertheless include opportunities for country-specific recognition and differentiated distribution of funds. In Fig. 1 , we propose a multilateral DSI benefit-sharing framework where access to DSI is “decoupled” from benefit-sharing from DSI. Benefit-sharing is ensured by mechanisms that do not limit access to DSI. This is a fundamental shift away from traditional control-oriented ABS to a new idea of OA (open access) and BS (benefit-sharing). This is necessary to protect the many benefits of openness and recognize that benefit-sharing can be accomplished without dramatically altering real-world access. New monetary mechanisms can be put into place upstream of DSI generation (e.g., a micro-levy on DSI-generation reagents and disposables), downstream of DSI use (e.g., a user fee on bio-based products), and/or outside the DSI life cycle (e.g., payment from high-income nation international development funds). To achieve simplicity, benefit-sharing must be based upon the entire global DSI dataset and not on individual sequences. This reflects the science: analysis of sequences can only be done by comparing them to all other DSI and, thus, have zero value in isolation. Fundamental bioinformatic techniques, like sequence alignment, search, and annotation, are founded on this comparative principle. We caution, however, against paywalls which, although simple and understandable, would not qualify as open access and would fundamentally break the interoperability of data in the current DSI ecosystem. In our model, the DSI data ecosystem itself would remain virtually the same for the user and would need only modest behind-the-scenes adaptation to generate funds. To incentivize the generation of biodiversity data, funds would be distributed via project-based applications based on a country’s development status and their DSI contribution to the global dataset. Those LMICs that contribute more DSI to the global dataset (by providing access to genetic resources), would receive comparatively more funds. This would create an incentive to illuminate biodiversity blind spots and build up in-country expertise, thereby creating a positive feedback loop. Notably, such a system could also be expanded to other international fora that are debating DSI such as the International Treaty on Plant Genetic Resources for Food and Agriculture, the World Health Organization, and the UN Convention on the Law of the Sea potentially yielding a “harmonized” solution. For this system to work, the scientific community needs to improve practice with regard to recording the country of origin for DSI and correct legacy problems. At present, only 16% of sequences in the INSDC have country of origin information associated with them; 44% of sequences without country data could and should have had country information provided by the submitting scientists [7] . Geographical information is not only important for policymakers, but it is also useful scientific data that should be reported as a matter of scientific integrity and the FAIR principles, which place a strong emphasis on the importance of reliable “provenance” metadata [12] . Importantly, the INSDC recently announced a new policy ( https://www.insdc.org/spatio-temporal-annotation-policy-18-11-2021 ) requiring spatio-temporal information demonstrating their commitment to scientific transparency and openness to change. Challenges still remain. For example, sequences that are listed in a patent application often have country information listed in the patent application. Although these same sequences are automatically submitted to the INSDC by patent offices, the country information is not transferred. This remains a significant loss of transparency given the fact that patent-associated DSI represents 20% of the INSDC dataset [7] . Nevertheless, scientific databases are not regulatory entities. They are scientific infrastructures with a public mission. In our view, they can play a supportive role in the policy process by providing data to policymakers. As part of the Global Biodiversity Framework, DSI-holding databases could be called upon to coordinate and deliver “country reports”—global analysis of DSI submissions, user trends, capacity building and advancement on DSI provenance transparency (see above). These data could be linked back to the benefit-sharing calculation. Given that the INSDC is an American, European, and Japanese collaboration (all high-income countries and the US is a CBD observer), it would likely be advisable to work in close collaboration with a more diverse group of databases. Here, the increasingly active Global Biodata Coalition could play a leading role ( https://globalbiodata.org/ ). There remain unanswered questions such as how to ensure fairness to indigenous people and local communities in a multilateral system. This could be encouraged via a new data tag for indigenous people and local communities, for example [13] and simply making IPLCs directly eligible to receive monetary funds. It would also be counter-productive if users began to dump low-quality or repetitive DSI into the databases to “game” the system and artificially increase a country’s DSI proportion in the database. Here standards and internal quality checks would be essential and are actually realizable. Finally, economic modelling must be conducted to determine which of the monetary mechanisms listed above are most likely to be cost-effective, financially productive, and to minimize administrative costs. While all countries use and produce DSI, there remain significant inequalities. Practical issues ranging from more expensive access to molecular biological reagents, slower internet bandwidth that limits high-throughput analyses, financial limitations for research funding, limited bioinformatics training and career development opportunities, as well as brain drain, routinely limit those of us working in LMICs. Thus, any DSI benefit-sharing framework must support technical capacity building focused on genomics and bioinformatics. The goal should be to facilitate a “leapfrog” effect in which LMIC scientists are trained to exploit DSI even while inequalities in high-tech sequencing or laboratory infrastructure including technology transfer are still being addressed. With advances in cloud computing, open-source software, and open access DSI databases, the gaps are easier to fill than ever before if strategic investments are made. Science-focused capacity development within the CBD must be aimed both at conservation and building up the bioeconomy through sustainable use of bioresources. Local scientists and regional or national science academies should be involved in agenda-setting. Matchmaking platforms should be established that connect scientists across the globe and build up human capital enabling sustainable development. Decisions made at the Geneva meetings in March 2022 and, ultimately, at the 15th Conference of the Parties to the CBD later in 2022, will affect DSI practitioners for a generation to come. The crux of the decision will be whether governments want “control” over DSI through a bilateral system or whether they see the opportunity for greater scientific advancement and ultimately greater monetary value if they choose openness through a multilateral system. Given the importance of DSI for the scientific community, we call for policymakers to affirm multilateralism at the COP15 meeting and de-couple access to DSI from benefit-sharing—to break the “ABS” acronym into “OA” and “BS” where open access, benefit-sharing, capacity building, and biodiversity conservation thrive. We encourage policymakers to engage with their national DSI practitioners and with our Network to work together towards a thoughtful, workable and informed compromise.